Novel residues in avian influenza virus PB2 protein affect virulence in mammalian hosts Highly pathogenic avian H5N1 influenza viruses have sporadically transmitted to humans causing high mortality. The mechanistic basis for adaptation is still poorly understood, although several residues in viral protein PB2 are known to be important for this event. Here, we demonstrate that three residues, 147T, 339T and 588T, in PB2 play critical roles in the virulence of avian H5N1 influenza viruses in a mammalian host in vitro and in vivo and, together, result in a phenotype comparable to that conferred by the previously known PB2-627K mutation with respect to virus polymerase activity. A virus with the three residues and 627K in PB2, as has been isolated from a lethal human case, is more pathogenic than viruses with only the three residues or 627K in PB2. Importantly, H5N1 viruses bearing the former three PB2 residues have circulated widely in recent years in avian species in nature. Avian H5N1 influenza viruses pose a significant public health threat, as highlighted by their continued circulation in nature and their infection of humans with high mortality rates (386 deaths out of 650 confirmed cases as of 24 January 2014, according to http://www.who.int/ ). Several determinants of avian influenza viruses contribute to their virulence in and adaptation to mammalian hosts [1] , [2] , [3] , [4] , [5] , [6] . For example, the multiple basic amino acids in the hemagglutinin cleavage site are responsible for the systemic replication and virulence of highly pathogenic influenza viruses of the H5 and H7 subtypes in chickens and mice [2] , [7] . PB1-F2, encoded by the +1 reading frame of the PB1 segment, affects the virulence of H5N1 and pandemic 1918 viruses and is associated with the induction of cell death and severe secondary bacterial pneumonia [8] , [9] . NS1, which is an antagonist of the interferon-mediated antiviral host response, also contributes to influenza virus virulence [4] , [10] , [11] , [12] , [13] , [14] , [15] , [16] . The M1 protein influences the high virulence and replication of avian H5N1 influenza viruses in a mouse model [1] . Mutations in the nuclear export protein (NS2) of avian H5N1 viruses also contribute to enhanced polymerase activity in mammalian cells [17] . Among influenza virus proteins, however, PB2 is considered a major viral determinant for adaptation and virulence of avian viruses in mammals. For example, lysine at position 627 of PB2 (PB2-627K) is a key host-range determinant, being present in most seasonal human viruses, except for the current 2009 pandemic H1N1 viruses [18] , [19] , [20] . However, PB2-627K is not commonly present in avian influenza viruses, with the notable exception of the Qinghai Lake lineage of H5N1 viruses [21] , [22] . Moreover, the presence of PB2-627K, which was found in some H5N1 viruses isolated from humans in Hong Kong in 1997, correlates with high virulence in mice and allows these viruses to replicate efficiently in the upper respiratory tract of this mammalian host [2] , [6] . The D701N mutation in PB2 also caused the high pathogenicity of an avian H5N1 influenza virus in mice and its presence correlated with the adaptation of an avian H7N7 virus to mice [5] , [23] . The human virus-like residue PB2-271A enhanced the polymerase activity and replication of an influenza virus in mammalian cells [24] . In addition, arginine at position 591 of PB2, which is present in 2009 pandemic H1N1 viruses, confers efficient replication in mammals and compensates for the lack of the 627K and 701N adaptive mutations in this protein [25] , [26] . Although these mutations are important for the adaptation of influenza viruses to mammalian hosts, several H5N1 avian influenza viruses possess residues associated with low pathogenicity at these positions in PB2 yet exhibit high virulence in mammalian models, suggesting that these viruses use alternative strategies to replicate efficiently in their new mammalian hosts [27] , [28] , [29] , [30] . Here, we assess the polymerase activity, virus replication and pathogenicity of an avian H5N1 virus isolated in 2010 in Vietnam (with high pathogenicity in mice) and an earlier avian H5N1 virus (with low pathogenicity in mice), and identify new molecular determinants of virulence in mammals. Importantly, an H5N1 virus bearing these virulence-determining residues and 627K in its PB2 is more pathogenic than viruses with only the three residues or 627K in PB2; such a virus has been isolated from a lethal human case. Characterization of an avian H5N1 isolate from Vietnam The avian H5N1 A/duck/Vietnam/TY165/2010 (TY165) virus was isolated from the lungs of a dead duck collected in Vietnam in 2010. To characterize the pathogenicity of this virus in mammals, we determined the dose required to kill 50% of infected mice (MLD 50 ) and assessed its replication in mice. We found that this virus was highly pathogenic, replicating systemically in all organs tested and had an MLD 50 of 0.6 plaque-forming unit (p.f.u. 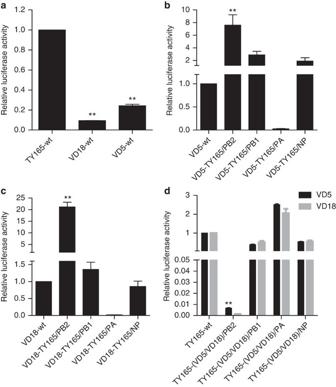Figure 1: Viral polymerase activity in human cells. Viral polymerase activity was determined by using mini-replicon assays in 293T cells. The data were normalized to wild-type TY165 (a,d), VD5 (b) and VD18 (c) levels. Polymerase activity of wild-type TY165, VD5 and VD18 replication complexes (a). Polymerase activity of wild-type and reassortant VD5 (b), VD18 (c) and TY165 (d) replication complexes. The data presented are the average of three independent experiments±s.d.Pvalues were calculated by using Student’st-test, **P<0.001. ; Table 1 ). Sequence analysis revealed that the virus possessed a polybasic amino acid stretch at the hemagglutinin cleavage site. 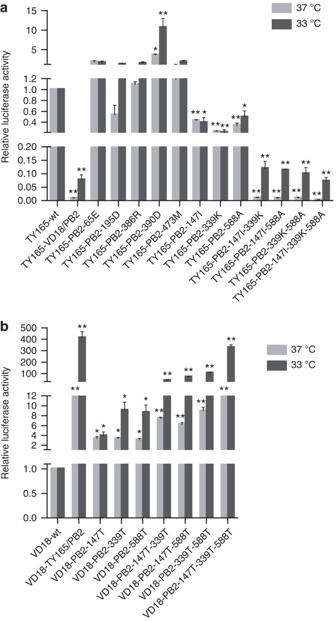Figure 2: Activity of wild-type and PB2 mutant polymerase complexes in human cells. The polymerase activity of wild-type and PB2 mutant TY165 (a) and VD18 (b) replication complexes was assessed in human 293T cells. Relative polymerase activities are shown for single, double and triple mutations in PB2 compared with wild-type levels. The data presented are the average of three independent experiments±s.d.Pvalues were calculated by using Student’st-test, comparing the polymerase activity of wild-type PB2 with that of the indicated mutant. **P<0.001; *P<0.05. However, its PB2, NS1 and PB1-F2 proteins did not have any known high pathogenicity-associated determinants ( Table 2 ) [2] , [5] , [11] , [23] , [25] , [26] . Table 1 The virulence and replication properties of two H5N1 viruses and their PB2 variants in BALB/ c mice. Full size table Table 2 Properties of the H5N1 viruses used in this study. Full size table The contribution of TY165-PB2 to the polymerase activity Although pathogenicity and host-range specificity of influenza viruses are polygenic traits, the polymerase is a determinant of these properties [2] , [5] , [6] , [18] , [24] , [25] , [26] , [31] . Therefore, we first compared the polymerase activity of TY165 with that of two avian H5N1 viruses with low pathogenicity in mice, A/chicken/Vietnam/NCVD5/2003 (VD5, with an MLD 50 value of more than 10 6 p.f.u.) and A/Muscovy duck/Vietnam/NCVD18/2003 (VD18, with an MLD 50 value of 10 4.3 p.f.u. ; Table 1 ), in human embryonic kidney 293T cells at 37 °C by using a mini-replicon assay. The polymerase complex of TY165 was significantly more active than that of VD5 or VD18 ( P <0.001, Student’s t -test; Fig. 1a ), suggesting that the polymerase complex of TY165 is better equipped to replicate in mammalian cells than is its counterpart in the low pathogenic avian strains of VD5 and VD18. To determine which component of the ribonucleoprotein complex (RNP; that is, PB2, PB1, PA or NP) contributes to the high activity of the TY165 polymerase, we tested the polymerase activity of RNPs composed of a variety of combinations of viral proteins from TY165, VD5 and VD18. We found that the PB2 protein of TY165 significantly increased the polymerase activity of both VD5 and VD18, by more than sevenfold and 20-fold, respectively ( Fig. 1b,c ). In contrast, the PB2 proteins of VD5 and VD18 substantially attenuated the polymerase activity of TY165 by as much as 142-fold and 1,000-fold, respectively ( Fig. 1d ). The PB1 protein of TY165 slightly enhanced the polymerase activity of VD5 and VD18, by about 2.6- and 1.3-fold, respectively, whereas the NP protein of TY165 marginally increased the polymerase activity of VD5, but decreased that of VD18 ( Fig. 1b,c ). The PA protein of TY165 downregulated the polymerase activity of VD5 and VD18 ( Fig. 1b,c ). Conversely, the PB1 and NP proteins of VD5 and VD18 slightly decreased the polymerase activity of TY165 (by less than twofold; Fig. 1d ). The PA proteins of both VD5 and VD18 enhanced the polymerase activity of TY165 ( Fig. 1d ). Our data thus show that the PB2 protein of TY165 significantly enhances the polymerase activity of the low pathogenic viruses VD5 and VD18, and that this effect is greater in the VD18 background. Since TY165-PB2 does not possess amino acid residues that are known to enhance polymerase activity in mammalian cells ( Table 2 ), this observation raises the possibility that as yet unknown molecular features in PB2 contribute to the high level of polymerase activity of TY165 in human cells. Figure 1: Viral polymerase activity in human cells. Viral polymerase activity was determined by using mini-replicon assays in 293T cells. The data were normalized to wild-type TY165 ( a , d ), VD5 ( b ) and VD18 ( c ) levels. Polymerase activity of wild-type TY165, VD5 and VD18 replication complexes ( a ). Polymerase activity of wild-type and reassortant VD5 ( b ), VD18 ( c ) and TY165 ( d ) replication complexes. The data presented are the average of three independent experiments±s.d. P values were calculated by using Student’s t -test, ** P <0.001. Full size image Three residues in PB2 cooperatively increase replication To identify amino acids in the PB2 protein of TY165 that contribute to its high polymerase activity in human cells, we compared the PB2 sequences between TY165 and VD18 or VD5. Of the 13 and 14 amino acid differences between TY165 and VD18 or VD5, respectively, the amino acid at positions 105, 108 and 369 in VD18 and 64, 81, 344 and 559 in VD5 were unique to these strains and appeared to be sporadic mutations. We therefore focused on the 10 amino acids (65E/D, 107S/N, 147I/T, 195D/N, 312K/R, 339K/T, 368R/Q, 390D/N, 473M/L and 588A/T) that were different between TY165 and VD18 or VD5 ( Table 2 ). These amino acids have not previously been linked to the pathogenicity of influenza viruses. We, therefore, singly introduced the eight residues 65E, 147I, 195D, 339K, 368R, 390D, 473M and 588A that were found in the low pathogenic virus into the PB2 of TY165; 107S and 312K were not tested because the former is highly variable and the latter is highly conserved among recent H5N1 isolates, which are highly pathogenic in mammalian species ( http://www.fludb.org/ ) [27] , [32] , [33] . We then performed mini-replicon assays in 293T cells at 33 °C (which is similar to the temperature of the upper respiratory tract in humans) and at 37 °C with these recombinant polymerase complexes and found that the polymerase activity of TY165 with each of the three residues (147I, 339K and 588A) was reduced by two- to fourfold under both temperature conditions ( Fig. 2a ). The introduction of these amino acids into TY165-PB2 in various combinations resulted in a substantial decrease in polymerase activity. To determine whether the three residues 147T, 339T and 588T in TY165-PB2 could increase the polymerase activity of VD18, we tested the polymerase activity of recombinant VD18 bearing PB2-147T, PB2-339T and PB2-588T singly or in combination and found that these residues increased the polymerase activity of VD18 ( Fig. 2b ). Of the VD18 PB2 mutants generated, the VD18 PB2 with all three mutations at positions 147, 339 and 588 exhibited the highest polymerase activity, which was comparable to that supported by TY165-PB2, suggesting that these three residues collectively contribute to viral polymerase activity ( Fig. 2a,b ). Figure 2: Activity of wild-type and PB2 mutant polymerase complexes in human cells. The polymerase activity of wild-type and PB2 mutant TY165 ( a ) and VD18 ( b ) replication complexes was assessed in human 293T cells. Relative polymerase activities are shown for single, double and triple mutations in PB2 compared with wild-type levels. The data presented are the average of three independent experiments±s.d. P values were calculated by using Student’s t -test, comparing the polymerase activity of wild-type PB2 with that of the indicated mutant. ** P <0.001; * P <0.05. Full size image Effect of three PB2 residues on virus growth in human cells To test the role of amino acids 147, 339 and 588 in PB2 on the replication of H5N1 viruses in human cells, we introduced mutations encoding the three low/high pathogenicity-associated residues (147I/T, 339K/T and 588A/T) into the PB2 segment of TY165 or VD18, generated mutant viruses by using reverse genetics (TY165-PB2-147I-339K-588A and VD18-PB2-147T-339T-588T), and compared the growth kinetics of the wild-type and mutant viruses in human airway epithelial Calu-3 cells at 33 or 37 °C. In these cells, TY165 replicated more efficiently than did VD18 by more than 1 log unit at 37 °C, although both viruses replicated to a similar level at 33 °C ( Fig. 3a,b ). The PB2-147T-339T-588T mutation markedly enhanced the replication of VD18 at all indicated time points at 37 °C ( Fig. 3c ). Similar results were obtained at 33 °C ( Fig. 3d ). Conversely, the replication of the TY165 mutant virus with PB2-147I-339K-588A was appreciably attenuated at both temperatures ( Fig. 3e,f ) with a more dramatic effect at 33 °C ( Fig. 3f ). These observations suggest that the combination of PB2 mutations at positions 147, 339, and 588 appreciably alters the replication of H5N1 viruses in mammalian cells, raising the possibility that these PB2 amino acids may also contribute to the high pathogenicity of TY165 in a mouse model. 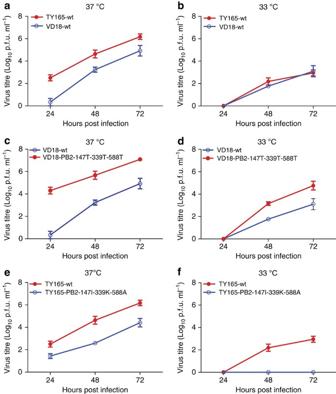Figure 3: Growth of viruses in Calu-3 cells at different temperatures. Growth of wild-type and mutant viruses in human Calu-3 cells infected at a multiplicity of infection of 10−4p.f.u. Growth of wild-type TY165 and VD18 viruses at 37 °C (a) and 33 °C (b). Growth of wild-type and mutant VD18 viruses at 37 °C (c) and 33 °C (d). Growth of wild-type and mutant TY165 viruses at 37 °C (e) and 33 °C (f). The data presented are the average of three transfection experiments carried out in parallel±s.d. from one experiment. Figure 3: Growth of viruses in Calu-3 cells at different temperatures. Growth of wild-type and mutant viruses in human Calu-3 cells infected at a multiplicity of infection of 10 −4 p.f.u. Growth of wild-type TY165 and VD18 viruses at 37 °C ( a ) and 33 °C ( b ). Growth of wild-type and mutant VD18 viruses at 37 °C ( c ) and 33 °C ( d ). Growth of wild-type and mutant TY165 viruses at 37 °C ( e ) and 33 °C ( f ). The data presented are the average of three transfection experiments carried out in parallel±s.d. from one experiment. Full size image Pathogenicity of PB2 reassortant viruses in mice To elucidate the contribution of the PB2 of TY165 to virulence and replication in a mammalian model, we determined the MLD 50 and replication in mice of PB2 reassortant viruses of VD18-TY165/PB2 (in which the PB2 segment of VD18 was replaced with the PB2 of TY165), TY165-VD18/PB2 (in which the PB2 of TY165 was replaced with the PB2 of VD18) and both wild-type VD18 and TY165 viruses. We found that replacement of VD18 PB2 with that of TY165 markedly enhanced the virulence of VD18 by more than 600-fold (MLD 50 of VD18-TY165/PB2 being 10 1.5 p.f.u. and that of VD18 being 10 4.3 p.f.u. ; Table 1 ). Although we did not detect replicating virus in any organs of mice infected with wild-type VD18 on day 3 post infection (p.i.) and detected only a low virus titre in the lungs on day 6 p.i. ( Table 1 ), high titres of VD18-TY165/PB2 were found in the lungs, nasal turbinates and spleen on day 3 p.i., and by day 6 p.i., the virus had spread to all other organs tested and was found at high titres. In contrast, the PB2 of VD18 attenuated TY165 by more than 1,000-fold (MLD 50 of wild-type TY165 being 0.6 p.f.u. and that of TY165-VD18/PB2 being 10 3.3 p.f.u. ; Table 1 ). In addition, TY165-VD18/PB2 was found only in the lungs on day 3 p.i., and in the lungs and spleen with a low titre on day 6 p.i., whereas wild-type TY165 replicated systemically in all organs tested on day 6 p.i. ( Table 1 ). Together, these data indicate that the PB2 of TY165 contributes to its high virulence and systemic replication in mice. Pathogenicity of PB2 mutant viruses in mice Next, we examined the contribution of the PB2 amino acids at positions 147, 339 and 588 to virulence in mice. First, we infected mice with viruses possessing single mutations in the TY165 background (TY165-PB2-147I, TY165-PB2-339K and TY165-PB2-588A). We found that the single mutations had no appreciable effect on the virulence of TY165, resulting in MLD 50 values comparable to that of wild-type virus ( Table 1 , Supplementary Fig. 1a ). Likewise, a TY165 virus possessing the PB2-147I-339K double mutation (tested because viruses with mutations at these positions are frequently found in nature; see below) caused weight loss in infected mice and resulted in an MLD 50 value comparable to that of the parental TY165 virus ( Table 1 , Supplementary Fig. 1a ). However, the triple mutant virus TY165-PB2-147I-339K-588A was markedly attenuated with an MLD 50 value of 10 2.8 p.f.u. ( Table 1 , Supplementary Fig. 1a ). Also, unlike wild-type TY165 and the PB2-147I-339K double mutant, the mutant virus TY165-PB2-147I-339K-588A replicated only in the lungs at 3 days p.i., and in the lungs and spleen with low titres at 6 days p.i. ( Table 1 ). Since the individual mutations at positions 147, 339 or 588 did not appreciably affect the weight loss and survival of the infected animals, we did not determine the virus titres in the organs of the animals infected with these variants. These data show that the triple mutation PB2-147I-339K-588A decreased the virulence and replication of TY165 in mice, which is consistent with our polymerase activity and growth kinetics data in human cells. Next, we tested whether PB2-147T, -339T and/or -588T enhanced the pathogenicity and replication of VD18: Viruses possessing the PB2-147T, -339T or 147T-339T mutations were comparable to the parental VD18 virus in terms of MLD 50 values and the extent of weight loss experienced by the infected mice ( Table 1 , Supplementary Fig. 1b ). Infection of mice with the VD18-PB2-558T mutant resulted in an MLD 50 value of 10 3.3 p.f.u., compared with an MLD 50 value of 10 4.3 p.f.u. for VD18 ( Table 1 ). In contrast, the triple VD18-PB2-147T-339T-588T mutant exhibited high virulence with an MLD 50 value of 10 1.5 p.f.u. compared with 10 4.3 p.f.u. for the VD18 wild-type virus ( Table 1 , Supplementary Fig. 1b ). Wild-type VD18 replicated only in the lungs with a low titre on day 6 p.i. ( Table 1 ); the PB2-147T-339T double-mutant replicated to higher titres than the wild-type virus in the lungs and low virus titres were also detected in the spleen on day 6 p.i. ( Table 1 ). In contrast, the mutant VD18 virus with PB2-147T-339T-588T was present at appreciably higher titres in the lungs and spread to the nasal turbinates, spleen, kidney and brain. These data show that the high pathogenicity-associated PB2-147T, -339T and -588T amino acids jointly contribute to the high virulence and systemic replication of TY165 in mice. Phylogenetic analysis of H5N1 PB2 sequences To assess the inheritance of PB2-147T, -339T and -588T, we phylogenetically analysed the PB2 sequences of H5N1 viruses in the so-called goose/Guangdong lineage of H5N1 viruses circulating since 1996. H5N1 PB2 nucleotide sequences were obtained from GenBank ( http://www.ncbi.nlm.nih.gov ) and GISAID ( http://platform.gisaid.org ). We added the PB2 sequence from A/chicken/Scotland/1959 as an outgroup. To obtain accurate ancestral inferences, we analysed only sequences that do not lack more than 100 amino acids at either end of the PB2 protein sequence. Duplicate sequences from the same strain and sequences with questionable amino acid translations were removed. The final data set contained 2,552 PB2 sequences, with 586 and 1966 sequences from GISAID and GenBank, respectively. The PB2 segment of TY165 (shown in Fig. 4 ) is genetically closely related to that of other duck viruses isolated in Vietnam in 2011 and 2012; these viruses also contain the three residues that we determined in this study to be associated with high pathogenicity (that is, 147T, 339T and 588T in PB2) (coloured in red in Fig. 4 ). Interestingly, all strains bearing the three high pathogenicity residues (147T, 339T and 588T) belong to a lineage that can be distinguished from the so-called Qinghai Lake viruses [21] , [34] , [35] (shown in dark blue in Fig. 4 ). Viruses in the Qinghai Lake lineage possess 147T and 339T, together with the known pathogenicity marker PB2-627K, which TY165 and the ‘red-coloured’ viruses lack. Our analysis indicates that these two groups (that is, the ‘red-coloured’ and ‘blue-coloured’ viruses) have common ancestors that first acquired the 339T mutation (coloured in sea blue in Fig. 4 ) and then the 147T mutation. Viruses possessing the PB2-147T-339T mutations (coloured in green in Fig. 4 ) then evolved into two separate lineages with the PB2-627K or -588T mutations. 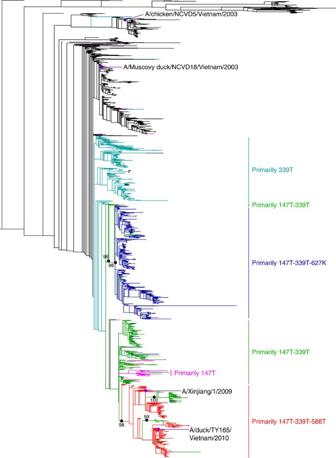Figure 4: Phylogenic relationships of the PB2 genes of H5N1 viruses. Colours indicate viruses primarily encoding PB2-147T (pink); -339T (sea blue); -147T-339T (green); -147T-339T-588T (red); -147T-339T-627K (dark blue, Qinghai Lake viruses); viruses not encoding any of the pathogenicity markers at positions 147, 339, 588 or 627 are shown in black. Also shown are the viruses used in this study (A/duck/TY165/Vietnam/2010, A/chicken/NCVD5/Vietnam/2003, A/Muscovy duck/NCVD18/Vietnam/2003) and A/Xinjiang/1/2009 (see text). Bootstrap support for topological details relevant to the emergence of these four pathogenicity markers are indicated with a black bullet when this support exceeds 70%; the actual bootstrap support is given next to the bullet. Figure 4: Phylogenic relationships of the PB2 genes of H5N1 viruses. Colours indicate viruses primarily encoding PB2-147T (pink); -339T (sea blue); -147T-339T (green); -147T-339T-588T (red); -147T-339T-627K (dark blue, Qinghai Lake viruses); viruses not encoding any of the pathogenicity markers at positions 147, 339, 588 or 627 are shown in black. Also shown are the viruses used in this study (A/duck/TY165/Vietnam/2010, A/chicken/NCVD5/Vietnam/2003, A/Muscovy duck/NCVD18/Vietnam/2003) and A/Xinjiang/1/2009 (see text). Bootstrap support for topological details relevant to the emergence of these four pathogenicity markers are indicated with a black bullet when this support exceeds 70%; the actual bootstrap support is given next to the bullet. Full size image To further assess the history of the 147T, 399T and 588T amino acids found in the TY165-PB2 protein, we determined the frequency by year of these three markers in the dataset described above. We found that the most ancestral pathogenicity marker, PB2-339T, increased in frequency around 2002–2003, resulting in a significant percentage (~40%) of strains possessing PB2-339T (while encoding low pathogenicity markers at PB2-147 and -588; Fig. 5a , upper left). The next pathogenicity marker, PB2-147T, increased in frequency from 2005 onwards, thus yielding appreciable numbers of viruses containing the high pathogenicity markers PB2-147T and -339T (but encoding a low pathogenicity marker at PB2-588; Fig. 5a , upper right). Viruses containing PB2-147T-339T were the ancestors of the Qinghai Lake viruses, which emerged in 2005; Qinghai Lake viruses encode the high pathogenicity marker PB2-627K in addition to PB2-147T-339T ( Fig. 5a , lower left). Viruses encoding PB2-147T-339T also founded the new lineage described here (encoding PB2-147T-339T-588T), which represents more than 50% of the available H5N1 sequences since 2011 ( Fig. 5a , lower right). 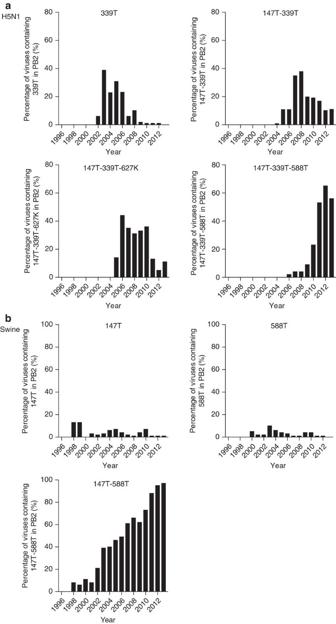Figure 5: Percentages of viruses possessing high pathogenicity-associated residues at amino acid positions 147, 339 and/or 588 of PB2. Amino acid sequences of the PB2 proteins of influenza viruses were analysed. The percentages per year of H5N1 (a) and swine (b) viruses containing the indicated combinations of high pathogenicity-associated amino acids 147T, 339T and/or 588T in their PB2 are shown. Figure 5: Percentages of viruses possessing high pathogenicity-associated residues at amino acid positions 147, 339 and/or 588 of PB2. Amino acid sequences of the PB2 proteins of influenza viruses were analysed. The percentages per year of H5N1 ( a ) and swine ( b ) viruses containing the indicated combinations of high pathogenicity-associated amino acids 147T, 339T and/or 588T in their PB2 are shown. Full size image Next, we asked whether the novel virulence markers identified here are comparable to the effect of 627K with respect to virus polymerase activity. We compared the polymerase activity of polymerase complexes bearing the three high pathogenicity-associated residues PB2-147T, -339T and -588T with a polymerase complex possessing 627K in the VD18 background by using the mini-replicon assay at 33 and 37 °C. We found that the polymerase activity of VD18 with the three novel residues in PB2 was similar to that of the virus with the 627K mutation alone at 37 °C ( Fig. 6a,b ), although at 33 °C, the polymerase activity of the virus with the 627K mutation was higher than that of the virus with the three novel residues ( Fig. 6b ), indicating that 147T, 339T and 588T are comparable to the effect of 627K at least at 37 °C. 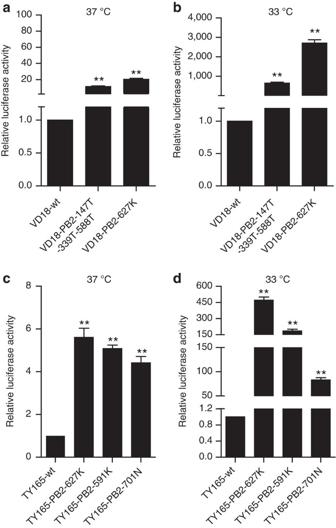Figure 6: Effects of PB2 pathogenicity determinants on viral polymerase activity. Viral polymerase activity in mini-replicon assays in 293T cells was compared among wild-type and variants possessing 147T/339T/588T or 627K (a,b). Viral polymerase activity in mini-replicon assays in 293T cells was compared among wild-type and variants possessing 627K, 591K or 701N (c,d). The data presented are the average of three independent experiments±s.d.Pvalues were calculated by using Student’st-test, comparing the polymerase activity of wild-type PB2 with that of the indicated mutant. **P<0.001. Figure 6: Effects of PB2 pathogenicity determinants on viral polymerase activity. Viral polymerase activity in mini-replicon assays in 293T cells was compared among wild-type and variants possessing 147T/339T/588T or 627K ( a , b ). Viral polymerase activity in mini-replicon assays in 293T cells was compared among wild-type and variants possessing 627K, 591K or 701N ( c , d ). The data presented are the average of three independent experiments±s.d. P values were calculated by using Student’s t -test, comparing the polymerase activity of wild-type PB2 with that of the indicated mutant. ** P <0.001. Full size image Combined effect of new pathogenicity markers and PB2-627K To assess whether 591K, 627K or 701N together with the three high pathogenicity-associated PB2 mutations we identified here could further enhance the replicative ability of an H5N1 virus in human cells, we evaluated the effect of PB2-147T, -339T and -588T with the mutation PB2-591K, 627K or 701N on polymerase activity in the TY165 backbone at 33 and 37 °C, that is, we introduced these mutations into TY165-PB2. We found that each of these mutations increased the polymerase activity of TY165, and that the effect was more dramatic at 33 °C than at 37 °C ( Fig. 6c,d ). Among the mutations tested, PB2-627K had the strongest effect. These findings suggest that acquisition of PB2-591K, -627K or -701N for viruses that already possess PB2-147T, -339T and -588T may create viruses with high replicative ability in mammals, including humans. To test the above possibility in vivo , we generated TY165 (possessing PB2-147T, -339T and -588T), TY165-PB2-147I-339K-588A-627K and TY165-PB2-627K (possessing PB2-147T,-339T,-588T and -627K) viruses. Because TY165 is already highly pathogenic in BALB/ c mice (MLD 50 =0.6 p.f.u. ), we would not expect to see any increase in virulence even if PB2-627K enhanced its virulence. We therefore tested the virulence of these mutant viruses in Mx1 +/+ mice, which carry Mx1 alleles; the Mx protein confers resistance to influenza infection [36] , but is not functional in most laboratory mouse strains, including BALB/ c . We found that TY165 and TY165-PB2-147I-339K-588A-627K did not kill Mx1 +/+ mice even at the high dose of 10 4 p.f.u. ; however, the TY165-PB2-627K virus was highly lethal to Mx1 +/+ mice at a dose of less than 5.6 p.f.u., although all of these viruses showed similar high pathogenicity in BALB/ c mice ( Table 3 ). Table 3 The virulence and replication properties of TY165 and mutant variants in Mx1 +/+ mice. Full size table On day 3 p.i., the TY165-PB2-627K and TY165-PB2-147I-339K-588A-627K viruses efficiently replicated in the lungs, nasal turbinates and spleens of Mx1 +/+ mice, whereas TY165 only replicated in the lungs and was recovered from the nasal turbinates of only one animal and at a lower virus titre ( Table 3 ). On day 5 p.i., the TY165-PB2-627K and TY165-PB2-147I-339K-588A-627K viruses replicated to comparable titres ( Table 3 ). These results indicate that the amino acids at positions 147, 339 and 588 of PB2 do not only affect viral replication and transcription, but additional functions which are currently unknown; for example, the amino acids at positions 147, 339 and 588 may affect the interaction of PB2 with host components involved in responses to influenza virus infection. Consequently, virus titres of the TY165-PB2-147I-339K-588A-627K and TY165-PB2-627K viruses are comparable, but their virulence in Mx1 +/+ mice differs. Our data thus demonstrate that H5N1 viruses containing these three new high pathogenicity-associated PB2 amino acids in combination with PB2-627K display substantially higher pathogenicity than viruses with only the three new pathogenicity-associated amino acids or PB2-627K alone. Here, we identified three amino acids, 147T, 339T and 588T, in PB2 that are critical for efficient replication and high virulence of an H5N1 influenza isolate, TY165, in mammalian cells. H5N1 viruses with these three PB2 residues have been circulating in nature over the last 4 years ( Figs 4 and 5 ). Furthermore, introduction of PB2-627K into an H5N1 virus with PB2-147T, -339T and -588T increased its pathogenicity, as demonstrated in Mx1 +/+ mice ( Table 3 ). An H5N1 virus with all four pathogenicity-associated PB2 amino acids (A/Xinjiang/1/2009; H5N1; indicated in Fig. 4 ) was isolated from a 31-year-old woman in 2009 in China who succumbed to her infection [37] . Collectively, these data demonstrate the threat that H5N1 viruses encoding PB2-147T-339T-588T may pose to human health. Mutations in the polymerase complex are critical for influenza viruses to adapt and infect new host species [19] , [30] , [36] , [37] ; notable examples of such mutations include 271A, 627K, 701N and 591R/K in PB2 (refs 2 , 3 , 5 , 6 , 17 , 20 , 22 , 24 , 25 , 30 ). Here, we identified additional mutations in PB2 which affect virulence, namely, 147T, 339T and 588T. A contribution to virulence of individual amino acid changes at position 147, 339 or 588 of PB2 has been reported [24] , [38] , [39] , [40] : three studies compared PB2-588T (typically found in avian influenza virus PB2 proteins) with PB2-588I (the amino acid commonly found in human influenza virus PB2 proteins) and reported increased viral polymerase activity for PB2-588I in mammalian cells [24] , [38] , [40] . However, these studies did not assess the significance of PB2-588A versus PB2-588T, as tested here. Liu et al. [39] reported that a PB2-339K to PB2-339T mutation reduced the cap-binding activity of PB2 and virulence in mice, while increasing replicative ability in MDCK cells. In contrast, we did not detect differences in mouse virulence between viruses encoding PB2-339T or PB2-339K. This difference may be explained by the genetic background of the viruses used. An M-to-L mutation at position 147 of a PB2 protein derived from an H9N2 virus increased virulence [41] , demonstrating a contribution of PB2-147 to virulence. However, these previous studies did not test the PB2-147T, -339T and -588T mutations in concert. Here, we demonstrate that 147T, 339T and 588T act together to affect H5N1 virus virulence; specifically, we found that the overall effect of the three combined mutations is greater than the sum of the individual effects on virulence. For example, the MLD 50 values of the TY165 and VD18 single and double mutants are comparable to the MLD 50 values of the parental viruses (with the exception of the VD18-PB2-588T mutation, which reduces the MLD 50 value by one log unit compared with the wild-type virus), whereas the MLD 50 values of the triple mutant viruses increased or decreased by about three log units ( Table 1 ). This cooperative effect is also reflected in the survival rates ( Supplementary Fig. 1 ); for example, all mice infected with 10 2 p.f.u. of the TY165-PB2-147I, -339K or -588A viruses succumbed to their infections, as did the mice infected with 10 2 p.f.u. of the TY165-PB2-147I-339K double mutant. In contrast, all mice infected with 10 2 p.f.u. of the TY165-PB2-147I-399K-588A triple mutant virus survived their infections. Our findings emphasize that there exist multiple genetic constellations (such as PB2-627K or PB2-147T-339T-588T) that may render viruses highly virulent. Moreover, functional interactions among different sites as described here add significant complexity to the potential prediction of virulence-enhancing mutations. The two H5N1 viruses we studied here, TY165 isolated in 2010 and VD18 isolated in 2003, are not genetically closely related ( Fig. 4 ); yet, the introduction of the three mutations into VD18 made it highly pathogenic ( Table 1 ). Therefore, our findings indicate that these amino acids in PB2 likely have a broad effect on virulence. What function(s) are affected by mutations at position 147, 339 and 588 of PB2? An X-ray crystallographic model shows that the residue at position 339 is located in the PB2 cap-binding domain (amino acids 318–438) and is near 357H, 361K, 376K and 404F, which modulate cap-binding and regulate transcription ( Supplementary Fig. 2a ) [42] . A recent study reported that a mutation from Lys to Thr at position 339 of PB2 affected cap-binding activity [39] . The amino acid at position 588 in the carboxyl-terminal domain of PB2 is close to residues 591 and 627, which are responsible for high pathogenicity in mammalian models ( Supplementary Fig. 2b ) [2] , [25] (Protein Data Bank accession codes 2VQZ and 3KC6 ). No structural information is available for residue 147 of PB2. The answer to the above question and the exact mechanism by which the amino acids at positions 147, 339 and 588 of PB2 affect the adaptation of avian H5N1 influenza viruses to mammalian hosts currently remain unknown. Interestingly, we found that a high percentage of swine influenza viruses encoding PB2-147T-588T (which were associated with increased polymerase activity in this study) has circulated since 1998 ( Fig. 5b ; lower left). In particular, about 80% of North American swine viruses acquired both mutations by 2011. In contrast, the percentage of swine viruses encoding only one of these markers, that is, PB2-147T ( Fig. 5b , upper left) or PB2-588T ( Fig. 5b , upper right) has remained low. Because the PB2 gene of the 2009 pandemic H1N1 viruses originated from a North American swine influenza virus, almost all of the 2009 pandemic H1N1 viruses have the high pathogenicity-associated residues of 147T and 588T in their PB2 ( http://www.fludb.org/ ). The high pathogenicity-associated residues 147T and 588T, together with PB2-591R/K (refs 25 , 26 ), may, therefore, have supported the ability of swine viruses to circulate in nature and paved the way for the 2009 pandemic H1N1 viruses to replicate efficiently in humans. In this study, we also found that TY165 PB1 slightly increased the polymerase activity of the VD5 and VD18 replication complexes. On the other hand, the PA segment of TY165 decreased the polymerase activity of the VD5 and VD18 viruses. The mechanisms and biologic significance of the effects of TY165 PB1 and PA on the replicative ability of other H5N1 viruses require further investigation. Cells MDCK cells (obtained from ATCC) were maintained in Eagle’s minimal essential medium (MEM) containing 5% newborn calf serum and antibiotics. Human embryonic kidney 293T cells (obtained from ATCC) were grown in Dulbecco’s modified essential medium (DMEM) with 10% fetal calf serum and antibiotics. Human airway epithelial cells (Calu-3, obtained from Raymond Pickles, University of North Carolina, Chapel Hill, NC) were cultured in DMEM/F12 supplied with 10% fetal calf serum with antibiotics. All cells were maintained at 37 °C with 5% CO 2 unless otherwise stated. Viruses The H5N1 A/duck/Vietnam/TY165/2010 (H5N1, TY165) virus used in this study was isolated from a sample collected in Vietnam in 2010. The A/chicken/Vietnam/NCVD5/2003 (H5N1,VD5) and A/Muscovy duck/Vietnam/NCVD18/2003 (H5N1,VD18) viruses have been previously described [6] , [43] ( Table 2 ). All H5N1 viruses used in this study were generated by using reverse genetics and were amplified in 10-day-old embryonated chicken eggs in a biosafety level 3 containment laboratory approved for such use by the Centers for Disease Control and Prevention and the US Department of Agriculture. Plasmid construction and reverse genetics The cDNAs of the TY165 virus were synthesized by reverse transcription of viral RNA with an oligonucleotide (Uni12), as previously described [2] . These cDNAs were then amplified by using PCR with gene-specific oligonucleotide primers and cloned into the pPolI vector for viral RNA production [44] . The reverse genetics systems for VD5 and VD18 are described elsewhere [6] , [19] , [43] . The PB2 pPolI mutant constructs were produced by site-directed mutagenesis PCR with primers that possessed the desired mutations [1] . All primer sequences used in this study are provided in Supplementary Table 1 . For viral protein expression constructs, whole segments of PB1, PA, NP and wild-type and mutant PB2s of all viruses were inserted into the pCAGGS/BsmBI vector. All constructs were sequenced to ensure the absence of unwanted mutations. The TY165, VD18 and VD5 viruses were produced by means of reverse genetics as described by Neumann et al. [44] . The reporter gene plasmid pPol-VD5(50)M(50)-Luc was used to produce negative-sense RNA containing the 3′ non-coding region and 50 nucleotides of the 3′ coding region of the M vRNA, the firefly luciferase gene and 50 nucleotides of the 5′ coding region and the 5′ non-coding region of the M vRNA. This construct was generated as follows: the fragment was amplified by using the back-to-back primers BsmBI-F977 (5′-CACACACGTCTCCGGGTGGTCATTTTGTCAACATAGAA-3′) and BsmBI-R50 (5′-CACACACGTCTCCGGGTTTCGACCTCGGTTAGAAGAC-3′) from the pPol plasmid containing the VD5 M gene and was incubated with BsmBI. The Luc gene was then cloned into the BsmBI site. Mouse experiments Four- to 6-week-old female BALB/c mice (Jackson Laboratory, Bar Harbor, ME) and 6- to 8-week-old female Mx1 +/+ mice (provided by Drs Peter Staeheli and Otto Haller, University of Freiburg, D-79104 Freiburg, Germany) were used for these experiments. To determine the dose required to kill 50% of infected mice (MLD 50 ), three mice per group for each virus were anaesthetized with isoflurane and inoculated intranasally with 10-fold serially diluted virus in a 50-μl volume. The mice were monitored daily for 14 days and checked for changes in body weight and mortality. The mice were killed if they lost more than 25% of their initial body weight. For virus replication in organs, groups of mice (six mice per group) were infected intranasally with 10 3 p.f.u.. Three mice in each group were killed on days 3 and 6 p.i., respectively. Organs (brains, lungs, nasal turbinates, kidneys and spleens) were collected for virus titration by use of plaque assays in MDCK cells. The data shown are the mean virus titres±s.d. Mini-replicon assay 293T cells were transfected with 0.25 μg each of the pCAGGS [45] constructs encoding the polymerase protein PB1, PA, NP and wild-type or mutant PB2, together with 0.05 μg of the mini-genome of pPol-VD5(50)M(50)-Luc (which encodes the firefly luciferase gene) and 0.025 μg of pGL4.74[hRluc/TK] (an internal control, Promega, Madison, WI). The transfected cells were incubated at 33 or 37 °C. At 48 h post transfection, the cells were lysed and the luciferase activity was determined by using the dual-luciferase system detector kit according to the manufacturer’s protocol (Promega). The luciferase activity values were normalized to the Renilla activity. The data presented are the average of three independent experiments±s.d. Virus replication in Calu-3 cells Confluent human airway epithelial Calu-3 cells were infected with wild-type or mutant H5N1 viruses at a multiplicity of infection of 10 −4 , and incubated for 1 h at 37 °C. After the 1 h incubation, the cells were washed twice and then further incubated in MEM/F12 containing 0.3% bovine serum albumin and TPCK trypsin (2.0 μg ml −1 ) at 33 and 37 °C. Aliquots of supernatants were collected for virus titration at 24, 48 and 72 h p.i.. Virus titres at each time point were determined by use of plaque assays in MDCK cells. Values are presented as the average of three independent experiments±s.d. Phylogenetic analysis PB2 gene sequences of highly pathogenic H5N1 influenza viruses of the goose/Guangdong lineage from avian, mammalian and other natural hosts were drawn from Genbank and GISAID. Sequences from laboratory mutants were excluded from the sample. Only PB2 sequences that do not lack more than 100 amino acids at either end were retained in the analysis. Duplicate sequences from the same strain and sequences with questionable amino acid translations were removed. This selection process resulted in a dataset of 2,552 sequences, including the PB2 sequence from A/chicken/Scotland/1959 for an outgroup. Sequences were aligned using CLUSTALW [46] , then edited manually as needed. RAxML [47] on CIPRES [48] was used to infer a phylogeny for the final dataset, using the GTR model of evolution with a gamma model of rate heterogeneity; 100 bootstrap replicates under this model were used to assess topological certainty. The final tree ( Fig. 4 ) was displayed in Archaeopteryx [49] . Biosafety This study was approved by the local Institutional Biosafety Committee and evaluated by NIAID who concluded that this study does not involve Dual Use Research of Concern (DURC). Ethics Our experiments in mice followed the University of Wisconsin-Madison’s Animal Care and Use Protocol. They were approved by the Animal Care and Use Committee of the University of Wisconsin-Madison (protocol number V00806), which acknowledged and accepted both the legal and ethical responsibility for the animals, as specified in the Fundamental Guidelines for Proper Conduct of Animal Experiment and Related Activities in the Animal Welfare Act and associated Animal Welfare Regulations and Public Health Service Policy (USA). How to cite this article : Fan, S. et al. Novel residues in avian influenza virus PB2 protein affect virulence in mammalian hosts. Nat. Commun. 5:5021 doi: 10.1038/ncomms6021 (2014).